Dynamic switching between escape and avoidance regimes reducesCaenorhabditis elegansexposure to noxious heat To survive, animals need to minimize exposure to damaging agents. They can either stay away from noxious stimuli (defined as avoidance), requiring the detection of remote warning cues, or run away upon exposure to noxious stimuli (defined as escape). Here we combine behavioural quantitative analyses, simulations and genetics to determine how Caenorhabditis elegans minimizes exposure to noxious heat when navigating in thermogradients. We find that worms use both escape and avoidance strategies, each involving the modulation of multiple parameters like speed and the frequency of steering and withdrawal behaviours. As some behavioural parameters promote escape while impairing avoidance, and vice versa, worms need to dynamically tune those parameters according to temperature. Furthermore, selectively disrupting avoidance or escape, through mutations affecting neuropeptide or TRPV channel signalling, increases exposure to heat. We conclude that dynamically switching between avoidance and escape regimes along the innocuous-noxious temperature continuum efficiently minimizes exposure to noxious heat. Motility is a central characteristic of animals and has probably been a critical drive for their success throughout evolution. Locomotion is essential for the most fundamental animal activities, including evading harmful situations. Here we consider two general behavioural responses aiming at reducing exposure to noxious agents: escape and avoidance. We define escape as behaviours directly triggered by exposure to noxious stimuli and used to run away from harmful situations. We define avoidance as behaviours used to stay away from deleterious situations. In this case, animals perceive warning signals and react before encountering a damaging agent. Efficient thermoregulation is required for animal growth and survival. For small ectotherms, which temperature rapidly equilibrate with surrounding environments, thermoregulation is prominently achieved through locomotion [1] , [2] . Although noxious heat or cold may directly trigger escape behaviours [3] , temperature cues may also serve as a warning signal driving avoidance behaviours. The small nematode Caenorhabditis elegans is a useful model to address the neurobiological mechanisms controlling behaviour [4] , [5] , [6] , [7] . Worm crawling behaviour is of low complexity and can be objectively quantified with computer-assisted analyses [8] . Worms move forward or backward by producing sinusoidal undulations of their body and make turns. Turns have been classified as omega-turns, where worms make a pronounced bending of their body (to look like the Greek letter omega, Ω) [9] , [10] , or as shallow turns (or steering), where worms produce gentler reorientations [11] , [12] , [13] . Worms can grow and reproduce in a ~13–26 °C temperature range. When crawling in spatial thermogradients covering this innocuous temperature range, worms accumulate around a preferred temperature, which depends on the past conditions of cultivation [1] , [14] , [15] . Depending on their position in the gradient, animals use negative thermotaxis to move toward lower temperatures, positive thermotaxis to move toward higher temperatures and isothermal tracking to remain close to their preferred temperature [2] , [11] , [16] , [17] . Negative thermotaxis is particularly robust in well-fed worms and has been extensively studied [1] , [2] , [16] , [18] . It involves a biased-random walk, consisting in periods of forward locomotion (runs), interrupted by punctual reorientation events (turns) [18] . During negative thermotaxis, worms adjust their turning probability (and consequently run duration) by monitoring the temporal changes in temperature created by their self-movement in the gradient. At a given temperature, worm turning probability is high when temperature rises and low when temperature decreases, leading to a drift down temperature gradients. By analogy to its definition in the field of thermodynamics [19] , we will use here the term ‘thermal hysteresis’ to describe the property of behaviours that differ upon heating or cooling over a given temperature range. In addition to thermotaxis occurring over innocuous temperatures, worms also display behaviours that are specific to noxious temperatures (above ~26 °C). When forward moving animals encounter a local noxious heat source, they produce a stereotyped withdrawal response, consisting in the following steps: stop, reversal to backward locomotion for one to two body lengths, omega turn and restart of forward locomotion in a new direction [20] , [21] . In addition, heat stimuli targeting animals’ tail cause them to accelerate [22] . It is not known to what extent these acute escape behaviours contribute to longer range navigation in thermogradients, neither how these responses are integrated with other avoidance mechanisms. Here we used quantitative behaviour analyses, computer simulations and genetic analyses with mutant animals to decipher how C. elegans minimizes exposure to noxious heat. In particular, we wanted to know how animals integrate avoidance and escape strategies when navigating in thermogradients. Our data show that escape and avoidance strategies are sustained by specific, yet partially counteracting behavioural mechanisms; are controlled by separate signalling pathways; and promote efficient thermoregulation provided that key behavioural parameters are dynamically tuned according to the thermal context. We propose similar mechanisms might be engaged in other organisms and in response to other stimuli, which intensity covers an innocuous-noxious continuum. Worms use multiple heat-evoked behavioural mechanisms In order to define the behavioural strategies used by worms to reduce exposure to noxious heat, we recorded movies of worms crawling at constant temperatures, exposed to heating and cooling temporal ramps ( Supplementary Fig. S1a,c ), or moving in spatial thermogradients ( Supplementary Fig. S1b,d ). Those movies were analysed with a tracking software [23] to quantify behaviour as a function of temperature and of temperature changes. To abolish the confounding effect of negative thermotaxis behaviours, we used wild-type adult worms starved for more than 5 h, a treatment known to suppress thermotactic responses [1] (see Supplementary Note 1 ). First, we evaluated the instant speed of worms in the 20–32 °C range upon heating, cooling or at constant temperature. Consistent with prior reports [1] , we found that worm average speed increases with temperature ( Fig. 1a , Supplementary Table S1 ). There was, however, a significant shift in the speed–temperature relationship in heating versus cooling ramps. Between 21 and 26 °C, worms moved faster upon cooling than upon heating ( Fig. 1a ). Speed values at constant temperature were not significantly different from those in the cooling situation ( Supplementary Table S1 ). A similar speed thermal hysteresis effect was also observed in spatial thermogradients ( Fig. 1b–d ), where animals moving down the gradient (toward cooler temperatures) moved significantly faster than animals moving up the gradient (toward higher temperatures). 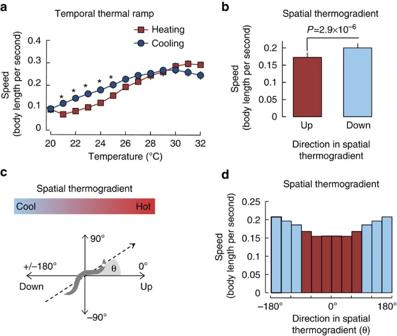Figure 1: Worms modulate speed according to temperature and temperature changes. (a) Wild-type (N2) worm speed was measured during heating (n=10) and cooling (n=10) temporal ramp assays and expressed as averages, with 95% confidence intervals as error bars. In each assay, 20–50 animals were tracked. Some error bars are smaller than the data points. Differences were assessed with a two-way ANOVA followed by Bonferronipost-hoctests (*P<.01). A thermal hysteresis effect is observed in the 21–26 °C range, where animals move faster upon cooling than upon heating. (b) Speed of animals measured in spatial thermogradient assays over the 24–28 °C range and expressed as averages, with s.e.m. as error bars (n=16 experiments). Worms moving up the gradient and down the gradient were compared. The difference was assessed by a two-tailed Student’st-test (theP-value is indicated on the figure). A significant thermal hysteresis effect is observed: animals move faster down the gradient (when self-movement causes cooling) than up the gradient (when self-movement causes heating). (c) Definition of the angleθof worm locomotion in a spatial thermogradient.θis set to 0° for worms facing the hot side of the gradient. (d) Details of the speed distribution as a function ofθfor the same set of experiments as described for panel (b). Figure 1: Worms modulate speed according to temperature and temperature changes. ( a ) Wild-type (N2) worm speed was measured during heating ( n =10) and cooling ( n =10) temporal ramp assays and expressed as averages, with 95% confidence intervals as error bars. In each assay, 20–50 animals were tracked. Some error bars are smaller than the data points. Differences were assessed with a two-way ANOVA followed by Bonferroni post-hoc tests (* P <.01). A thermal hysteresis effect is observed in the 21–26 °C range, where animals move faster upon cooling than upon heating. ( b ) Speed of animals measured in spatial thermogradient assays over the 24–28 °C range and expressed as averages, with s.e.m. as error bars ( n =16 experiments). Worms moving up the gradient and down the gradient were compared. The difference was assessed by a two-tailed Student’s t -test (the P -value is indicated on the figure). A significant thermal hysteresis effect is observed: animals move faster down the gradient (when self-movement causes cooling) than up the gradient (when self-movement causes heating). ( c ) Definition of the angle θ of worm locomotion in a spatial thermogradient. θ is set to 0° for worms facing the hot side of the gradient. ( d ) Details of the speed distribution as a function of θ for the same set of experiments as described for panel ( b ). Full size image Second, we evaluated the occurrence of withdrawal responses ( Fig. 2a ). Upon heating, the withdrawal probability rose progressively with temperature ( Fig. 2b ). In striking contrast, this behaviour was strongly suppressed upon cooling or at constant temperature, regardless of the temperature ( Fig. 2b , Supplementary Table S1 ). In spatial thermogradients, we also observed a strong increase of the withdrawal rate when worms were moving up the gradient as compared with down the gradient ( Fig. 2c ). We also evaluated the distribution of the reorientation angles upon withdrawal. For worms initially moving up the gradient (facing heat), the angle distribution was biased, with an enrichment in worms turning toward the opposite direction (90–180°) from their initial direction (before withdrawal onset; Fig. 2d ). In contrast, the rarer withdrawals made by worms moving down the gradient produced more random turns, with equal fractions of turns >90° and <90°. The bias was also observed upon heating in temporal ramps ( Fig. 2e,f ). Overall, our results show that worms upregulate their withdrawal rate upon heating and that these events preferentially reorient them away from heat. 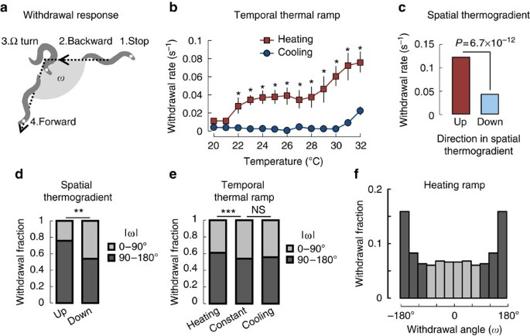Figure 2: Temperature and its changes affect withdrawal rate and reorientation angles. (a) Illustration of the withdrawal response showing the definition of the reorientation angleω. An animal, here initially moving toward the right side of the scheme, stops, reverses to backward locomotion and then undergoes an omega turn, before restarting forward locomotion in a new direction. The white dot labels the head of the animal. (b) Withdrawal rate measured during heating (n=10) and cooling (n=10) temporal ramp assays and expressed as averages, with 95% confidence intervals as error bars. In each assay, 20–50 animals were tracked. Some error bars are smaller than the data points. Differences were assessed with a two-way ANOVA followed by Bonferronipost-hoctests (*P<0.01). A thermal hysteresis effect is observed in the 22–32 °C range, where the withdrawal rate is higher upon heating than upon cooling. (c) Average withdrawal rate measured in spatial thermogradient assays over the 24–31 °C range. The number of withdrawals performed by worms moving up the gradient and down the gradient was compared. The difference was assessed by Fisher’s exact test (theP-value is indicated on the figure,n=253 withdrawal events). A significant thermal hysteresis effect is observed: animals perform significantly more turns when moving up the gradient (when self-movement causes heating) than down the gradient (when self-movement causes cooling). (d,e) The angle taken after withdrawals (ω) is influenced by the nature of the thermal stimuli. Withdrawal angle was analysed in spatial gradients (d), as well as in temporal thermal ramps (heating/cooling) and at constant temperature (e). Constant temperature data are aggregated from experiments at 25, 28 and 32 °C. **P=3.0 × 10−3byχ2-test (n=253 withdrawal events); ***P=1.4 × 10−3; NS, not significant (P=0.06) byχ2-test (n=3,379 withdrawal events). Angle indications correspond to absolute values. (f) Worms do not need spatial temperature differences to bias their turning after a withdrawal response. Detailed analysis of the angle taken during withdrawal events (ω) triggered by homogenous heating. The distribution is significantly different from a random model (P=5.0 × 10−28byχ2-test (n=2,064)). Figure 2: Temperature and its changes affect withdrawal rate and reorientation angles. ( a ) Illustration of the withdrawal response showing the definition of the reorientation angle ω . An animal, here initially moving toward the right side of the scheme, stops, reverses to backward locomotion and then undergoes an omega turn, before restarting forward locomotion in a new direction. The white dot labels the head of the animal. ( b ) Withdrawal rate measured during heating ( n =10) and cooling ( n =10) temporal ramp assays and expressed as averages, with 95% confidence intervals as error bars. In each assay, 20–50 animals were tracked. Some error bars are smaller than the data points. Differences were assessed with a two-way ANOVA followed by Bonferroni post-hoc tests (* P <0.01). A thermal hysteresis effect is observed in the 22–32 °C range, where the withdrawal rate is higher upon heating than upon cooling. ( c ) Average withdrawal rate measured in spatial thermogradient assays over the 24–31 °C range. The number of withdrawals performed by worms moving up the gradient and down the gradient was compared. The difference was assessed by Fisher’s exact test (the P- value is indicated on the figure, n =253 withdrawal events). A significant thermal hysteresis effect is observed: animals perform significantly more turns when moving up the gradient (when self-movement causes heating) than down the gradient (when self-movement causes cooling). ( d , e ) The angle taken after withdrawals ( ω ) is influenced by the nature of the thermal stimuli. Withdrawal angle was analysed in spatial gradients ( d ), as well as in temporal thermal ramps (heating/cooling) and at constant temperature ( e ). Constant temperature data are aggregated from experiments at 25, 28 and 32 °C. ** P =3.0 × 10 −3 by χ 2 -test ( n =253 withdrawal events); *** P =1.4 × 10 −3 ; NS, not significant ( P =0.06) by χ 2 -test ( n =3,379 withdrawal events). Angle indications correspond to absolute values. ( f ) Worms do not need spatial temperature differences to bias their turning after a withdrawal response. Detailed analysis of the angle taken during withdrawal events ( ω ) triggered by homogenous heating. The distribution is significantly different from a random model ( P =5.0 × 10 −28 by χ 2 -test ( n =2,064)). Full size image Third, we evaluated changes in trajectory caused by shallower turns (or steering) made during worm movement (see an example of this behaviour in Supplementary Movie 1 ). Steering events were flagged based on worm angular speed ( Fig. 3a ). As for withdrawal events, we observed a strong thermal hysteresis for the steering response ( Fig. 3b ). Upon heating, the steering rate rose from 20 to ~25 °C and then returned close to baseline over ~27 °C. In contrast, steering was strongly suppressed upon cooling at any temperature from 21–32 °C; leading to straighter trajectories as compared with the heating situation. The thermal hysteresis effect on steering was also observed in spatial thermogradients ( Fig. 3c ). The direction taken during steering events was not influenced by the gradient orientation. Indeed, favourable turns (leading worms to face lower temperatures) were as numerous as unfavourable turns (leading worms to face higher temperatures) ( Fig. 3d,e ). In addition, the distribution of the recorded angular speeds during steering was the same for favourable and unfavourable turns, in both cases with more shallow turns than sharp turns ( Fig. 3f ). These data suggest that worms do not modulate their steering direction according to the temperature gradient. Instead, worms increase the rate of steering as temperature rises to increase the chances they reorient away from heat, and suppress the rate of steering when temperature decreases to enable straight movement toward cooler temperatures. 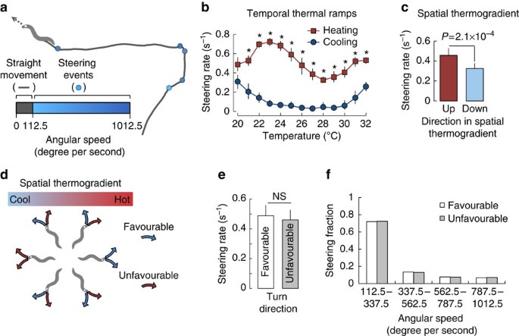Figure 3: Temperature and its changes affect steering rate but not steering direction. (a) Illustration of the steering response and of the steering event definition based on worm angular speed. See alsoSupplementary Movie 1. (b) Steering rate measured during heating (n=10) and cooling (n=10) temporal ramp assays and expressed as averages, with 95% confidence intervals as error bars. In each assay, 20–50 animals were tracked. Some error bars are smaller than the data points. Differences were assessed with a two-way ANOVA followed by Bonferronipost-hoctests (*P<0.01). A thermal hysteresis effect is observed in the 21–32 °C range, where the steering rate is higher upon heating than upon cooling. (c) Steering rate of animals measured in spatial thermogradient assays over the 24–28 °C range and expressed as averages, with s.e.m. as error bars (n=16 experiments). Worms moving up the gradient and down the gradient were compared. The difference was assessed by a two-tailed Student’st-test (theP-value is indicated on the figure). A significant thermal hysteresis effect is observed: the steering rate is lower for animals moving down the gradient (when self-movement causes cooling) than up the gradient (when self-movement causes heating). (d) Illustration of favourable and unfavourable turns. Favourable (resp. unfavourable) turns are defined as turns that lead to a reduction (resp. increase) in the time derivate of temperature caused by animal self-movement in the gradient. (e) Comparison of the rates of favourable and unfavourable steering events recorded for worms crawling in the 24–28 °C range of a spatial thermogradient. Data are expressed as averages, with s.e.m. as error bars (n=16 assays). NS, not significant by Student’st-test (P=0.70). (f) Comparison of the distributions of angular speed recorded during steering events for favourable and unfavourable turns. Figure 3: Temperature and its changes affect steering rate but not steering direction. ( a ) Illustration of the steering response and of the steering event definition based on worm angular speed. See also Supplementary Movie 1 . ( b ) Steering rate measured during heating ( n =10) and cooling ( n =10) temporal ramp assays and expressed as averages, with 95% confidence intervals as error bars. In each assay, 20–50 animals were tracked. Some error bars are smaller than the data points. Differences were assessed with a two-way ANOVA followed by Bonferroni post-hoc tests (* P <0.01). A thermal hysteresis effect is observed in the 21–32 °C range, where the steering rate is higher upon heating than upon cooling. ( c ) Steering rate of animals measured in spatial thermogradient assays over the 24–28 °C range and expressed as averages, with s.e.m. as error bars ( n =16 experiments). Worms moving up the gradient and down the gradient were compared. The difference was assessed by a two-tailed Student’s t -test (the P -value is indicated on the figure). A significant thermal hysteresis effect is observed: the steering rate is lower for animals moving down the gradient (when self-movement causes cooling) than up the gradient (when self-movement causes heating). ( d ) Illustration of favourable and unfavourable turns. Favourable (resp. unfavourable) turns are defined as turns that lead to a reduction (resp. increase) in the time derivate of temperature caused by animal self-movement in the gradient. ( e ) Comparison of the rates of favourable and unfavourable steering events recorded for worms crawling in the 24–28 °C range of a spatial thermogradient. Data are expressed as averages, with s.e.m. as error bars ( n =16 assays). NS, not significant by Student’s t -test ( P =0.70). ( f ) Comparison of the distributions of angular speed recorded during steering events for favourable and unfavourable turns. Full size image Collectively, our data show that worms use four behavioural mechanisms to reduce exposure to heat, which rely on modulating their speed, withdrawal rate, withdrawal angle and steering rate. Heat-evoked behaviours depend on short-term thermal history The thermal hysteresis properties highlighted above for speed, steering and withdrawal could depend either on instant changes in temperature, or on longer term thermal history. The progressive heating and cooling ramp experiments depicted above ( Supplementary Fig. S1c ) do not distinguish between the two possibilities. Indeed, at a given temperature (for example, 24 °C), animals in heating versus cooling ramps experience instant temperature changes, but have also very different temperature histories (20–24 °C for heating, 33–24 °C for cooling). Thus, we performed additional assays where worms (equilibrated around 24 °C) were exposed to rapid temperature rises or falls. Results showed a marked thermal hysteresis for speed, steering and withdrawal ( Supplementary Fig. S2 ). Thus, although not ruling out potential adaptation effects over longer time frames, our results show that short-term thermal history (in the range of seconds) is sufficient to account for the thermal hysteresis properties of speed, steering and withdrawal behaviours. Specific contributions of each mechanism In principle, the speed thermal hysteresis, the steering thermal hysteresis, the withdrawal thermal hysteresis and the withdrawal angle bias could each contribute to drive worms toward cooler temperatures. In order to weight those contributions, we created Monte-Carlo simulations of worm navigation in linear thermogradients. Animal speed, steering rate, steering angles, withdrawal rate and withdrawal angles were implemented to match the empirically measured distributions and to take into account the effect of temperature and its changes resulting from self-movement. We started with a full model integrating the four mechanisms. The shape of simulated trajectories was very similar to the one observed for real worms ( Fig. 4a ). Furthermore, we evaluated the ability of simulations to recapitulate long-range navigation in thermogradients by comparing empirical and simulated spatial distributions of worm populations after 60 min. Two distinct situations were compared: (i) the avoidance assay (starting temperature: 22 °C), where the ability of the worms to stay away from heat is assessed ( Fig. 4b ), and (ii) the escape assay (starting temperature: 30 °C), where the ability of the worms to run away from noxious heat is assessed ( Fig. 4c ). Although in the absence of gradient, worms largely dispersed over the plate (not shown), both empirical and simulated data show that worms efficiently stayed away from noxious heat in the avoidance assay and ran away from heat in the escape assay ( Fig. 4b,c ). Thus, our simulations recapitulate the most salient aspects of both avoidance and escape behaviours and can be used for further analyses. 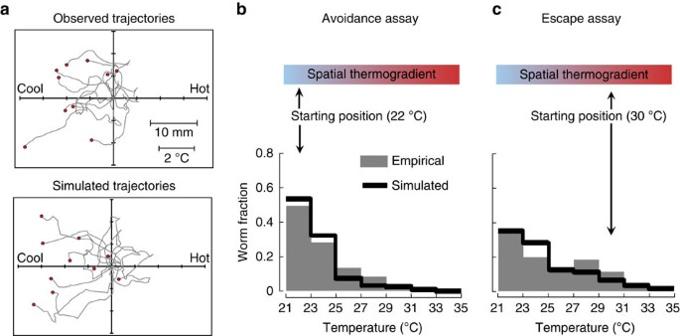Figure 4: Comparison of real versus simulated navigation of worms in spatial thermogradients. (a) Comparison of real and simulated trajectories recorded in a 2.7 °C cm−1gradient. For comparison purpose, starting coordinates were set at the axis intersection (0;0). Starting temperatures were in the 25–28 °C range. Tracks lasted 2–3 min and their ends are located with red dots. (b) Avoidance assay design and resulting empirical and simulated spatial distributions of worms. Worms started at 22 °C in a linear gradient from 21 to 35 °C (1.12 °C cm−1). The empirical distribution was recorded after 60 min of free crawling with real worms and is the average of four assays (each with more than 150 animals). The simulated distribution was determined with a model implementing all the identified mechanisms aiming at reducing heat exposure (n=500 animals). (c) Escape assay design and resulting empirical and simulated spatial distributions of worms. Worms started at 30 °C in a linear gradient from 21 to 35 °C (1.12 °C cm−1). The empirical distribution was recorded after 60 min of free crawling with real worms and is the average of four assays (each with more than 150 animals). The simulated distribution was determined with a model implementing all the identified mechanisms aiming at reducing heat exposure (n=500 animals). Figure 4: Comparison of real versus simulated navigation of worms in spatial thermogradients. ( a ) Comparison of real and simulated trajectories recorded in a 2.7 °C cm −1 gradient. For comparison purpose, starting coordinates were set at the axis intersection (0;0). Starting temperatures were in the 25–28 °C range. Tracks lasted 2–3 min and their ends are located with red dots. ( b ) Avoidance assay design and resulting empirical and simulated spatial distributions of worms. Worms started at 22 °C in a linear gradient from 21 to 35 °C (1.12 °C cm −1 ). The empirical distribution was recorded after 60 min of free crawling with real worms and is the average of four assays (each with more than 150 animals). The simulated distribution was determined with a model implementing all the identified mechanisms aiming at reducing heat exposure ( n =500 animals). ( c ) Escape assay design and resulting empirical and simulated spatial distributions of worms. Worms started at 30 °C in a linear gradient from 21 to 35 °C (1.12 °C cm −1 ). The empirical distribution was recorded after 60 min of free crawling with real worms and is the average of four assays (each with more than 150 animals). The simulated distribution was determined with a model implementing all the identified mechanisms aiming at reducing heat exposure ( n =500 animals). Full size image Next, we evaluated worm performances when some or all mechanisms were disabled. Simulations were run with starting temperatures ranging from 22–32 °C, and performances were assessed by measuring the end-point median temperature of worm populations after 60 min ( Fig. 5a ). From those data, we calculated a thermoregulation index (reflecting overall worm performances with the full range of starting temperatures), an avoidance index (reflecting performances with low starting temperatures) and an escape index (reflecting performances with high starting temperatures; see Methods). Disabling the four mechanisms systematically increased the end-point temperature and yielded very low thermoregulation, avoidance and escape indexes ( Fig. 5a,b ). 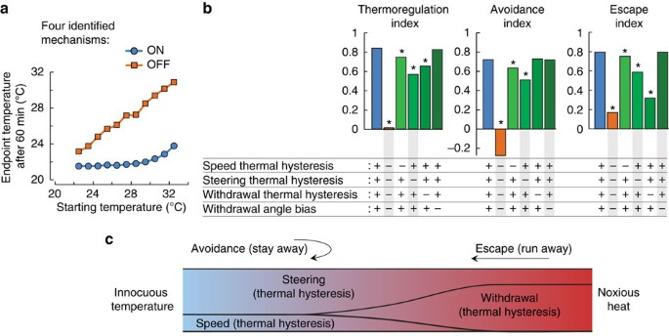Figure 5: Multiple mechanisms differentially contribute to worm avoidance and escape performances. (a) Simulation of worm long-range navigation in a linear gradient from 21 to 35 °C (1.12 °C cm−1). Starting temperatures were systematically varied to cover the innocuous-noxious range, from 22 to 33 °C. Worm performances were assessed by measuring the median end-point temperature reached by a population of 500 simulated animals after 60 min (as inFig. 4). Depicted results compare a full model implementing the four identified behavioural mechanisms (speed thermal hysteresis, steering thermal hysteresis, withdrawal thermal hysteresis and withdrawal angle bias) and a model where all of them are inactivated. (b) Simulations as in (a) were performed with selective inactivation of each of the four behavioural mechanisms, as indicated at the bottom of the graph. Thermoregulation, avoidance and escape indexes were calculated from the end-point temperatures experienced by worms after 60 min (see Methods). *P<0.001 versus full model (in blue) by Mann–WhitneyU-tests with Bonferroni corrections. (c) Schematic of the relative contributions of speed, steering and withdrawal thermal hysteresis to avoidance and escape performances along the innocuous-noxious range of temperature. Figure 5: Multiple mechanisms differentially contribute to worm avoidance and escape performances. ( a ) Simulation of worm long-range navigation in a linear gradient from 21 to 35 °C (1.12 °C cm −1 ). Starting temperatures were systematically varied to cover the innocuous-noxious range, from 22 to 33 °C. Worm performances were assessed by measuring the median end-point temperature reached by a population of 500 simulated animals after 60 min (as in Fig. 4 ). Depicted results compare a full model implementing the four identified behavioural mechanisms (speed thermal hysteresis, steering thermal hysteresis, withdrawal thermal hysteresis and withdrawal angle bias) and a model where all of them are inactivated. ( b ) Simulations as in ( a ) were performed with selective inactivation of each of the four behavioural mechanisms, as indicated at the bottom of the graph. Thermoregulation, avoidance and escape indexes were calculated from the end-point temperatures experienced by worms after 60 min (see Methods). * P <0.001 versus full model (in blue) by Mann–Whitney U -tests with Bonferroni corrections. ( c ) Schematic of the relative contributions of speed, steering and withdrawal thermal hysteresis to avoidance and escape performances along the innocuous-noxious range of temperature. Full size image In order to evaluate the respective contributions of the four mechanisms, we first disabled them one by one ( Fig. 5b ). Disabling the withdrawal angle bias did not cause detectable effects, but disabling each of the three thermal hysteresis-based mechanisms reduced worm thermoregulation performances. Disabling the speed thermal hysteresis markedly decreased the avoidance index. Disabling the withdrawal thermal hysteresis decreased only the escape index. Disabling the steering thermal hysteresis decreased both avoidance and escape indexes. Second, we performed simulations where each strategy is enabled alone ( Supplementary Fig. S3 ). Enabling only withdrawal thermal hysteresis strongly increased the escape index as compared with the situation where no mechanism is enabled. In contrast, enabling only speed or steering thermal hysteresis more markedly increased the avoidance index. Enabling only the withdrawal angle bias had no effect. Overall, our data indicate that worms primarily engage steering and speed thermal hysteresis-based mechanisms for noxious heat avoidance, while they mainly use a withdrawal thermal hysteresis-based mechanism to escape from noxious heat ( Fig. 5c ). Escape and avoidance mechanisms counteract Having shown that the thermal hysteresis of speed, steering and withdrawal is critical for worm thermoregulation, we wondered whether other behavioural parameters also have an influence. We pursued our simulations of navigation in thermogradients to systematically investigate the impact of the average worm speed and turning rate on the performances in avoidance assays (starting temperature: 22 °C) versus escape assays (starting temperature: 30 °C). For this set of simulations, we kept the thermal hysteresis unaltered, but varied the average speed and turning rate (both steering and withdrawal). This corresponds to keeping the cooling versus heating difference in the speed–temperature relationships ( Figs 1a , 2b , 3b ), but shifting both the cooling and heating curves up or down, around the empirically determined values. Our results show that as average speed increased, escape performances initially improved (with lower end-point temperatures), reached a plateau and then decreased (with higher end-point temperatures), while avoidance performances progressively decreased ( Supplementary Fig. S4a ). Increasing the turning rate improved worm avoidance performances to reach a floor effect, but it had the opposite effect in the escape assay ( Supplementary Fig. S4b ). These data illustrate the counteracting nature of behavioural mechanisms involved in avoidance and escape, respectively. Worms more efficiently stay away from heat with low speed and high turning rate, while they more efficiently run away with high speed and low turning rate ( Supplementary Fig. S4c ). Dynamic tuning of escape and avoidance mechanisms To achieve efficient thermoregulation in most situations, worms need both effective escape and avoidance mechanisms. Yet, as illustrated with simulation results ( Supplementary Fig. S4 ), escape and avoidance efficiency are antagonistically regulated by behavioural parameters such as speed and turning rate. This suggests that only sub-optimal overall thermoregulatory performances could be reached if those behavioural parameters were static. Instead, our data show that worms change those parameters according to temperature ( Figs 1 , 2 , 3 , and Supplementary Table S1 ). For example, as temperature rises from 22–28 °C, worms progressively increase their overall speed, but in parallel decrease their steering rate. This dynamic tuning phenomenon tends to improve escape at high temperature and avoidance at low temperature. To quantitatively evaluate the importance of the dynamic tuning effects, we created worm simulations where those effects are abolished by implementing constant values (averaged over the full-temperature range) for speed, steering and withdrawal rate. However, the overall thermal hysteresis was kept constant, that is, the average differences between cooling and heating situations were maintained. Our results show that fully suppressing the dynamic tuning on all three channels (speed, steering and withdrawal) substantially impaired worm behaviour, with higher end-point temperatures attained after 60 min of navigation ( Fig. 6a ). Next, we selectively disabled the dynamic tuning on each channel to evaluate their relative contribution ( Fig. 6b ). Disabling the dynamic tuning of speed had the strongest impact, decreasing both avoidance and escape indexes. Disabling the dynamic tuning of steering also had a negative impact on worm performances, but the magnitude of the effect was lower. Disabling the dynamic tuning of withdrawals slightly impaired escape performances, but improved avoidance performances, leading to a null net effect on the overall thermoregulation index. Collectively, those data indicate that worms improve thermoregulation through the dynamic tuning of speed, and to a lesser extent of steering, along the innocuous-noxious temperature continuum. 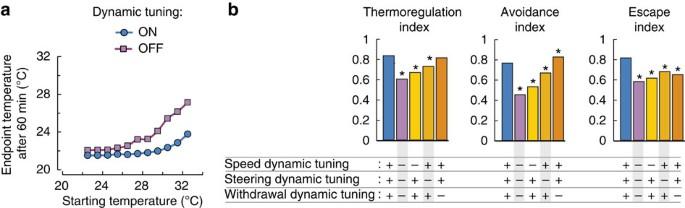Figure 6: Dynamic tuning of speed and steering along the innocuous-noxious temperature continuum improves worm thermoregulation. (a) Worm navigation in spatial gradient was simulated as inFig. 5. A full model (dynamic tuning: ON) was compared with a model where the overall temperature dependence of speed, steering and withdrawal is inactivated (dynamic tuning: OFF). The average thermal hysteresis was, however, maintained in the latter model. For each model, 5,500 trajectories were simulated (n=500 for each starting temperature). (b) Simulations as in (a) were performed with selective inactivation of the dynamic tuning affecting speed, steering and withdrawal, as indicated at the bottom of the graph. Thermoregulation, avoidance and escape indexes were calculated from the end-point temperatures experienced by worms after 60 min (see Methods). *P<0.001 versus full model (in blue) by Mann–WhitneyU-tests with Bonferroni corrections. Each thermoregulation index was derived from 5,500 simulated trajectories; each avoidance index was derived from 1,500 simulated trajectories; each escape index was derived from 1,500 simulated trajectories. Figure 6: Dynamic tuning of speed and steering along the innocuous-noxious temperature continuum improves worm thermoregulation. ( a ) Worm navigation in spatial gradient was simulated as in Fig. 5 . A full model (dynamic tuning: ON) was compared with a model where the overall temperature dependence of speed, steering and withdrawal is inactivated (dynamic tuning: OFF). The average thermal hysteresis was, however, maintained in the latter model. For each model, 5,500 trajectories were simulated ( n =500 for each starting temperature). ( b ) Simulations as in ( a ) were performed with selective inactivation of the dynamic tuning affecting speed, steering and withdrawal, as indicated at the bottom of the graph. Thermoregulation, avoidance and escape indexes were calculated from the end-point temperatures experienced by worms after 60 min (see Methods). * P <0.001 versus full model (in blue) by Mann–Whitney U -tests with Bonferroni corrections. Each thermoregulation index was derived from 5,500 simulated trajectories; each avoidance index was derived from 1,500 simulated trajectories; each escape index was derived from 1,500 simulated trajectories. Full size image Pleiotropic effects of mutations in TRPV and NPR-1 genes Mutations in the neuropeptide receptor-1 gene npr-1 , as well as in the TRPV channel genes ocr-2 and osm-9 affect worm distribution in noxious heat spatial thermogradient assays [24] , but the underlying behavioural mechanisms are not known. To gain more insight on the function of these genes, we compared the behaviour of mutants in heating and cooling ramps with that of wild-type animals. Our results highlight pleiotropic but distinct effects in animals harbouring the npr-1(ad609) mutation [25] or combining ocr-2(ak47) and osm-9(ky10) mutations [26] , [27] . First, we found that speed profiles were significantly affected in both mutants. Upon heating, the combined ocr-2 osm-9 mutations significantly reduced the maximum speed reached at high temperature, but did not affect baseline speed at 20 °C ( Fig. 7a ). Conversely, the npr- 1 mutation did not affect the maximal speed at high temperature, but significantly increased basal speed at 20 °C ( Fig. 7a ). Upon cooling, the ocr-2 osm-9 mutations reduced speed across the full-temperature range, whereas the npr-1 mutation had no effect ( Fig. 7b ). Consequently, the speed thermal hysteresis was reduced in both mutants ( Fig. 7c ). This implies that the two behavioural mechanisms based on speed dynamic tuning and on speed thermal hysteresis are impaired in each mutant, but due to different effects on the speed–temperature profiles. 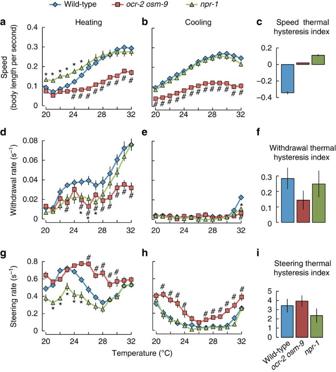Figure 7: TRPV channel and NPR-1 signalling have a pleiotropic impact on speed modulation, steering and withdrawal behaviours. npr-1(ad609)andocr-2(ak47)osm-9(ky10)mutants were compared with wild-type in temporal thermal ramp assays. (a,b,d,e,g,h) Speed, withdrawal and steering were assessed upon heating and cooling as inFigs 1a,2b,3b. Differences were assessed with two-way ANOVAs (temperature x genotype). We found significant genotype main effects for speed and steering upon heating and cooling and for withdrawals upon heating (F(38,455–468)=52.0 to 550.6,P<0.001), while the genotype effect was not significant for withdrawal upon cooling (F(38,455)=1.48,P=0.23). We found significant genotype × temperature interaction effects for speed and withdrawal upon heating and cooling, and for steering upon heating (F(38,455–468)=2.20 to 6.25,P<0.001), while the interaction effect was not significant for steering upon cooling (F(38,455)=1.33,P=0.14). ANOVAs were followed by Bonferronipost-hoctests. *P<0.05 between wild-type andnpr-1;#P<0.05 between wild-type andocr-2 osm-9. Data are expressed as means with s.e.m. as error bars. Some error bars are smaller than the data symbols. For all statistical comparisons,n≥10 experiments (each tracking 15 to 50 worms). (c,f,i) Thermal hysteresis indexes were calculated by subtracting the area under the curve (AUC) of the cooling curves from the AUC of the respective heating curves (ina,b,d,e,g,h). Considered temperature ranges were 20–28 °C for speed, 27–32 °C for withdrawal and 20–32 °C for steering. Units are °C body lenght s−1(c) and °C s−1(f,i). Figure 7: TRPV channel and NPR-1 signalling have a pleiotropic impact on speed modulation, steering and withdrawal behaviours. npr-1(ad609) and ocr-2(ak47)osm-9(ky10) mutants were compared with wild-type in temporal thermal ramp assays. ( a , b , d , e , g , h ) Speed, withdrawal and steering were assessed upon heating and cooling as in Figs 1a , 2b , 3b . Differences were assessed with two-way ANOVAs (temperature x genotype). We found significant genotype main effects for speed and steering upon heating and cooling and for withdrawals upon heating ( F (38,455–468) =52.0 to 550.6, P <0.001), while the genotype effect was not significant for withdrawal upon cooling ( F (38,455) =1.48, P =0.23). We found significant genotype × temperature interaction effects for speed and withdrawal upon heating and cooling, and for steering upon heating ( F (38,455–468) =2.20 to 6.25, P <0.001), while the interaction effect was not significant for steering upon cooling ( F (38,455) =1.33, P =0.14). ANOVAs were followed by Bonferroni post-hoc tests. * P <0.05 between wild-type and npr-1 ; # P <0.05 between wild-type and ocr-2 osm-9 . Data are expressed as means with s.e.m. as error bars. Some error bars are smaller than the data symbols. For all statistical comparisons, n ≥10 experiments (each tracking 15 to 50 worms). ( c , f , i ) Thermal hysteresis indexes were calculated by subtracting the area under the curve (AUC) of the cooling curves from the AUC of the respective heating curves (in a , b , d , e , g , h ). Considered temperature ranges were 20–28 °C for speed, 27–32 °C for withdrawal and 20–32 °C for steering. Units are °C body lenght s −1 ( c ) and °C s −1 ( f , i ). Full size image Second, we found that withdrawals were downregulated in both mutants upon heating ( Fig. 7d ), but unaffected upon cooling ( Fig. 7e ). More specifically, npr-1 mutation only impaired heat-induced withdrawals in the 25–27 °C range, while ocr-2 osm-9 mutations affected withdrawals more largely, with a very strong inhibition from 23–32 °C. The withdrawal thermal hysteresis is moderately affected in npr-1 mutant and more strongly affected in ocr-2 osm-9 mutant animals ( Fig. 7f ). Third, we found that steering was also profoundly modulated in both mutants. The mutation in npr-1 strongly decreased the steering response upon heating, in the 21–25 °C range ( Fig. 7g ), but not upon cooling ( Fig. 7h ), leading to a decrease in the steering thermal hysteresis index ( Fig. 7i ). The mutations in ocr-2 and osm-9 significantly upregulated steering, both upon heating and cooling ( Fig. 7g,h ), leaving the steering thermal hysteresis index close to wild-type values ( Fig. 7i ). The effects of single osm-9 and ocr-2 mutations on speed, steering and withdrawal were all significantly weaker than those of the double mutation ( Supplementary Fig. S5 ). These results suggest that osm-9 and ocr-2 work redundantly to control noxious heat-evoked behaviours. As a whole, our quantitative analyses of mutant behaviour highlight that signalling through NPR-1 and TRPV channels selectively controls several key behavioural mechanisms important for worm long-range navigation in noxious heat thermogradients. Separate control of escape and avoidance Based on simulations of worm navigation in thermogradients, we have proposed that distinct behavioural components specifically contribute to avoidance or escape behaviour performances ( Fig. 5c ). As mutations in npr-1 , ocr-2 and osm-9 genes differentially affect these behavioural components, they offer an opportunity to test this model. The mutation of npr-1 reduced the thermal hysteresis of speed and steering responses, but left intact the withdrawal response to high temperatures. This predicts that npr-1 mutants will retain good abilities to run away from heat, but be impaired in their ability to stay away from heat. In contrast, we found that combined mutations of ocr-2 and osm-9 genes markedly decreased heat-evoked withdrawal responses, while increasing overall steering rate and decreasing average speed. This predicts that ocr-2 osm-9 animals will retain good abilities to stay away from heat, but be impaired in their ability to run away from heat. To test these predictions, we first implemented the mutant deficits in our thermogradient navigation model. Quantitative data from these simulations confirmed our qualitative predictions ( Fig. 8a,b ). Next, we turned to real avoidance and escape assays (as in Fig. 4b,c ). In striking agreement with our predictions and simulated data, we found that npr-1 mutant animals were poor avoiders but good escapers, while ocr-2 osm-9 mutant animals were poor escapers but good avoiders ( Fig. 8c,d ). Collectively, these data indicate that performances in escape versus avoidance behaviours are controlled by genetically separable pathways. 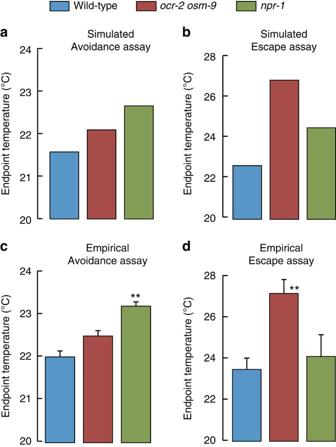Figure 8: NPR-1 promotes avoidance while TRPV channels promote escape. (a,b) Comparison of wild-type,npr-1andocr-2 osm-9mutants in thermogradient simulations, as inFig. 4, for the avoidance and escape assays. In each case, 500 worms were simulated for 60 min and the median temperature of the resulting worm distribution is reported. (c,d) Empirical data obtained in real worm population assays, as inFig. 4.n3 assays, each scoring at least 150 animals. Data are means with s.e.m. as error bars. One-way ANOVAs revealed significant differences across genotypes (avoidance:F(2,8)=18.09,P<0.01; escape:F(2,8)=9.29,P<0.01). **P<0.01 versus wild-type using Dunnet’spost-hoctests. Figure 8: NPR-1 promotes avoidance while TRPV channels promote escape. ( a , b ) Comparison of wild-type, npr-1 and ocr-2 osm-9 mutants in thermogradient simulations, as in Fig. 4 , for the avoidance and escape assays. In each case, 500 worms were simulated for 60 min and the median temperature of the resulting worm distribution is reported. ( c , d ) Empirical data obtained in real worm population assays, as in Fig. 4 . n 3 assays, each scoring at least 150 animals. Data are means with s.e.m. as error bars. One-way ANOVAs revealed significant differences across genotypes (avoidance: F (2,8) =18.09, P <0.01; escape: F (2,8) =9.29, P <0.01). ** P <0.01 versus wild-type using Dunnet’s post-hoc tests. Full size image Our data show that the navigation of worms in noxious heat thermogradients implicates several mechanisms: First, worms engage withdrawal-associated reorientations. By upregulating withdrawals upon heating but suppressing them upon cooling (thermal hysteresis), worms lengthen runs toward cooler temperatures and shorten runs toward higher temperatures. Similar biased-random walks are used by many organisms in a variety of goal-directed behaviours, like chemotaxis [10] , [28] , phototaxis [29] or thermotaxis [18] , [30] . Although the mechanism of negative thermotaxis engaged in innocuous temperatures relies on turns of random orientation [18] , withdrawal angles produced upon noxious heat stimulation are non-random and animals tend to turn toward cooler temperatures. This behaviour thus relates to the ‘pirouette’ mechanism in worm chemotaxis, where animals tend to orientate toward the peak of chemo-attractant [10] , [13] . However, our simulation results indicate that this withdrawal angle bias has a relatively modest contribution to worm performances in thermogradients, and might be more important for acute escape from very local heat sources. Second, worms use steering to produce smoother reorientations. This type of behaviour has been described in the weathervane mechanisms of chemotaxis [13] and during isothermal tracking [11] , [18] . In these latter behaviours, turn directions are directly influenced by the gradient orientation. In contrast, in noxious heat thermogradients, the direction of turns is not influenced by the orientation of the gradient. However, because the turning events during steering are subject to thermal hysteresis, they function as the motile force for a biased-random walk mechanism. Thus, worms combine two distinct biased-random walks: one using withdrawal-associated sharp turns and the other using steering events. Third, worms modulate their speed to move faster upon cooling and slower upon heating. The speed shift resulting from this thermal hysteresis effect is sufficient to drive worms toward cooler temperatures. Indeed, even with a constant turning rate, runs of equal duration up or down the gradient will cover longer distances toward cool temperatures than toward high temperatures. In addition, worms adjust their average speed according to temperature (speed dynamic tuning). If speed was constant over the full temperature range, then wild-type worms would be either good escapers but bad avoiders (with high speed), or good avoiders but bad escapers (with low speed). Dynamically adjusting the locomotory output according to the thermal environment circumvents this limitation. Speed modulation behaviours have previously been documented in response to acute events, like the slowing of worms that enter food or that are exposed to low O 2 tensions, and have been proposed to contribute to navigation in oxygen gradients [31] , [32] . However, to our knowledge, our study is the first quantitative analysis of speed modulation as a determinant of worm long-range, goal-directed navigation. Our data showed that avoidance and escape behaviours are not only conceptually distinct, but are executed in mechanistically and genetically separable ways. Some fundamental behavioural parameters (such as speed, discussed above) involved in both avoidance and escape manoeuvres have counteracting effects on worm thermoregulation performances. Such counteracting drives suggest that a single mechanism could not by itself ensure good performances in avoidance and escape behaviours, actually providing an explanation for the existence of several complementary mechanisms. Yet, even with multiple mechanisms available, worms cannot engage them all at the same time because they partially neutralize each other. To circumvent this intrinsic limitation, worms dynamically tune some critical parameters (like speed and steering rate) according to temperature. By this mean, worms favour efficient heat avoidance mechanisms when they are within innocuous temperatures and favour efficient escape mechanisms when they are exposed to noxious heat. This behavioural transition presents some similarities with the local search/dispersal behavioural switch observed following food deprivation [33] and to the dwelling/roaming switches regulated by the quality of food and associated with optimal foraging strategies [34] , [35] , [36] . Thus, changing the behavioural rules according to environmental inputs is not only important to improve foraging and exploratory behaviours, but also help minimizing the exposure to noxious heat. In conclusion, the present study provides insights on the necessity of balancing escape and avoidance strategies, as well as on their underlying behavioural mechanisms. Further studies are now made possible in C. elegans to investigate the molecular and neural mechanisms involved. In addition, there is no reason to believe that the efficacy of dynamic tuning mechanisms should be limited to temperature-related behaviours, nor to C. elegans . Thus, we presume that similar mechanisms involving a well-coordinated avoidance/escape transition, might be engaged in other species and in response to various stimuli, which intensity covers an innocuous-noxious continuum (for example, chemicals, pH, osmolarity and O 2 tensions), in order to minimize exposure to damaging agents and to improve survival. Worm maintenance and starvation Worm strains were the following: wild-type (N2), CX10 osm-9(ky10) IV, CX4544 ocr-2(ak47) IV, LX748 ocr-2(ak47) osm-9(ky10) IV [37] and DA609 npr-1(ad609) X. Animals were maintained according to standard cultivation protocols on nematode growth medium (NGM) agar plates [38] . For all experiments, we used first-day adult hermaphrodite animals that had been starved for 5–8 h, as described previously [24] . Heating and cooling temporal ramps We constructed a Peltier element-based device for heat stimuli delivery. Square (4 cm × 4 cm) 72W Peltier elements were sandwiched between a GPU waterblock cooling unit (Aquatuning, Germany) and a square aluminium plate (7.5 cm × 7.5 cm × 1.5 mm). Water, maintained at 24±1 °C, circulated at 4 l min −1 into the waterblock. Current in the Peltier element was controlled with a Proportional Integrative Derivative (PID) controller (McShane Inc., USA). Temperature feedback was recorded with a small thermistor taped to the aluminium plate. Before the assay, worms were washed from the starvation plate with distilled water, centrifuged 1 s with a mini centrifuge at full-speed (MyFuge Mini, Biolabo Scientific Instruments SA, Switzerland), and the re-suspended animal pellet (10 μl) was deposited inside a glycerol coral on a 6 cm NGM plate. The glycerol coral was made by cutting a 3 mm large frame in Whatman paper, socking it in 60% glycerol, and depositing it on the top of the assay plate. The internal dimensions of the coral were 2.5 cm × 1.7 cm. A small thermistor was placed at the top of the agar surface and maintained under the glycerol coral. This thermistor was used to record the actual agar surface temperature before and during the thermal ramps. Starting temperatures averaged 20.0 °C (s.d.=0.1) for heating ramps and 33.1 °C (s.d.=0.3) for cooling ramps. Comparison of baseline temperatures for heating and cooling experiments, across the three examined genotypes by one-way analyses of variance (ANOVAs) revealed no significant difference (heating: F (2,34) =2.11, P =0.14; cooling: F (2,35) =2.93, P =0.07). To ensure reproducible thermal stimuli across experiments, each assay plate was weighted to finely adjust the heating/cooling power. The heating slopes (measured in the linear range from 23–33 °C) averaged 0.186 °C s −1 (s.d.=0.015) and the cooling slopes (measured in the linear range from 30–22 °C) averaged −0.181 °C s −1 (s.d.=0.014). Comparison of the slopes across the three examined genotypes by one-way ANOVAs revealed no significant differences (heating: F (2,34) =2.65, P =0.09; cooling: F (2,35) =1.86, P =0.17). Thus, genotype-associated differences reported in the Result section cannot be accounted for by any systematic variations in the baseline temperature or in the delivered temperature stimuli. Rapid thermal stimuli For the thermal stimuli reported in Supplementary Fig. S2 , starved animals were equilibrated for 5 min at 23 or 25 °C and were submitted to a rapid thermal heating or cooling, respectively. The resulting thermal slopes (mean heating slope=0.190 °C s −1 , s.e.m.=0.011; mean cooling slope=−0.191 °C s −1 , s.e.m.=0.012) were similar to those measured in the heating and cooling temporal ramps described above. To achieve a nearly instant thermal acceleration with minimal mechanical stimulations for the worms, a chunk of NGM-agar from the pre-equilibration plate was quickly but smoothly transferred on the top of a pre-heated (34 °C) or pre-cooled (14 °C) aluminium plate. Linear thermal slopes were achieved within 2–3 s ( Supplementary Fig. S2a ), allowing behavioural comparisons for symmetrical thermal stimuli around 24 °C (heating from 23.5–24.5 °C; cooling from 24.5–23.5 °C) as depicted in Supplementary Fig. S2b,c,d . Thermogradient assays Temperature gradients were generated as previously described [24] . For movie recordings, a 2.7±0.2 °C cm −1 linear gradient was generated in 6 cm diameter NGM petri dishes. Movie recordings lasted 6 min and no coral was used. For long-range thermogradient assay, a 1.1±0.1 °C cm −1 linear gradient was generated in rectangular 12.5 cm × 7.5 cm petri dishes. Movie recordings Worms were illuminated obliquely with a square of red light emitting diodes (LED), constructed with two DIODER four-piece light strip sets (Ikea, Switzerland). The heated aluminium plate was covered with a black tape for dark field imaging. We used a Navitar 7010 Macro-zoom (Videal, Switzerland) coupled to a 640 × 480 pixel, DMK 21BU04.H USB camera (The Imaging Source, Germany) to record movies as .avi files. Frame rate was 7.5 frames per second. For thermal ramps, the field of view was 1.71 cm × 1.28 cm in size and centred in the middle of the coral to avoid recording animals performing glycerol-evoked behaviours when reaching the coral borders. For thermogradients, the field of view was 3.10 cm × 2.33 cm in size, covering a region from ~24 to ~31 °C. Movie analyses Movies were analysed off-line with the Multi-Worm Tracker software [23] . For each frame, the software identifies objects (animals) and records the coordinates of their centres of mass, the coordinates of an eleven point skeleton matching each animal, as well as animal length (linearly measured from one object extremity to the other) and width (linearly measured perpendicularly to the length axis). Objects were tracked over the full movies. We used custom-designed spreadsheets to compute raw data and extract the relevant behavioural parameters. All data were smoothed on a five frame interval (centred moving average of the centre of mass coordinates, as well as of the skeleton coordinates). Tracks terminated when worms moved out of the field or upon worm collision. To remove potential artefacts caused by these events and by the data smoothing with moving averages, we removed the data corresponding to the first 10 and last 10 frames of each track. The detailed procedure to evaluate speed, steering event probability and withdrawal event probability is described in the Supplementary Methods and Supplementary Fig. S6 . Number of tracking experiments and statistics For each genotype and for each thermal ramp or gradient protocol, we analysed at least 10 different worm preparations (each with between 15 and 50 animals tracked) during experiments performed on at least three different days. We used SPSS (IBM) to perform Student’s t -tests and ANOVAs. The χ 2 and Fisher’s exact tests were performed for discrete event contingency comparisons (calculated with R from the BiostaTGV interface http://marne.u707.jussieu.fr/biostatgv/ ). Data fitting were done thanks to the http://zunzun.com/ platform. Computer behavioural simulations Worm locomotion in linear thermogradients was simulated using custom written spreadsheets and Visual Basic macros. For each simulation, 500 animals were run sequentially. Animals were considered as punctual objects evolving in a 12.5 cm long ( x axis) and 7 cm large ( y axis) dish, with a linear thermogradient from 21 to 35 °C along the x axis. Animals started at defined positions in the gradient: x coordinate was manipulated to match the desired starting temperature, while y coordinate was randomized. Their initial direction was random. Animals reaching the dish border were set to restart locomotion perpendicularly to the border. Animal coordinates were refreshed at intervals of one second and monitored over 60 min. For every time interval, animals did three things: (1) they moved according to their precedent direction for a distance defined by their speed (a new position was then defined); (2) they decided whether to do a withdrawal; (3) they decided whether to do a steering event. At every position, the speed magnitude was defined according to an empirical data-based speed–temperature profile and corrected for thermal hysteresis effects. Similarly, the probabilities of withdrawal and steering event occurrence were defined according to empirical data-based withdrawal rate-temperature and steering rate-temperature profiles and corrected for thermal hysteresis effects. Details on the simulation unfolding and on the model mathematical development are presented in Supplementary Methods , Supplementary Data 1 , and Supplementary Figs S7,S8,S9 . Calculation of Avoidance and Escape indexes A Performance score was calculated as follows: Performance score=( T start − T reached )/( T start − T minimun ) T start is the imposed starting temperature in the simulation, T reached is the median end-point temperature reached by the population after 60 min, and T minimun is the minimum temperature that could have been reached by animals (21 °C). A positive performance score indicates that worms have moved toward cooler temperature relative to their starting temperature, whereas a negative score indicates they have moved toward higher temperatures. The thermoregulation index was calculated as the average performance score for starting temperatures homogeneously spread over the 22–33 °C range. The Avoidance index was obtained with the same calculation, but over the 22–24 °C range. The Escape index was obtained with the same calculation, but over the 30–33 °C range. How to cite this article: Schild, L. C. and Glauser, D. A. Dynamic switching between escape and avoidance regimes reduces Caenorhabditis elegans exposure to noxious heat. Nat. Commun. 4:2198 doi: 10.1038/ncomms3198 (2013).